A small molecule modulates Jumonji histone demethylase activity and selectively inhibits cancer growth The pharmacological inhibition of general transcriptional regulators has the potential to block growth through targeting multiple tumorigenic signalling pathways simultaneously. Here, using an innovative cell-based screen, we identify a structurally unique small molecule (named JIB-04) that specifically inhibits the activity of the Jumonji family of histone demethylases in vitro , in cancer cells, and in tumours in vivo. Unlike known inhibitors, JIB-04 is not a competitive inhibitor of α-ketoglutarate. In cancer, but not in patient-matched normal cells, JIB-04 alters a subset of transcriptional pathways and blocks viability. In mice, JIB-04 reduces tumour burden and prolongs survival. Importantly, we find that patients with breast tumours that overexpress Jumonji demethylases have significantly lower survival. Thus, JIB-04, a novel inhibitor of Jumonji demethylases in vitro and in vivo , constitutes a unique potential therapeutic and research tool against cancer, and validates the use of unbiased cellular screens to discover chemical modulators with disease relevance. Over the last years, evidence has accumulated demonstrating the widespread deregulation of transcription factors and histone-modifying enzymes in cancer [1] , [2] , [3] , [4] , [5] , [6] . Conceptually, the hijacking of these general regulators by the oncogenic process can give tumours a greater survival advantage and wider environmental response flexibility than co-opting a specific protein that acts within a single cascade. As a corollary, inhibition of such general regulators has the potential to block growth through targeting multiple tumorigenic signaling pathways simultaneously, a scenario that could also diminish the development of resistance. Currently available chemical modulators of drugable transcription factors and epigenetic enzymes include ligands of nuclear hormone receptors [7] , inhibitors of myc/max dimerization [8] , metal chelators that neutralize the active-site zinc in histone deacetylases (HDACs) [9] , [10] , and modulators of proteins with other histone-modifying activities [11] , [12] , [13] , [14] , [15] . Recent work in cancer drug discovery has focused on the development of competitive analogues of co-factors that modulate the activity of epigenetic enzymes upregulated in tumours, such as the Jumonji-C-containing histone demethylases that control transcriptional programmes through the modulation of lysine methylation. These efforts have identified several promising candidates with inhibitor activity in purified systems [16] , [17] , [18] , [19] , and in some cases, cell-permeable compounds have been described with high micromolar or millimolar potencies in culture [20] , [21] , [22] , [23] . None of these co-factor analogues have yet been shown to possess biological activity in animal models. We set out to identify structurally unique, selective chemical modulators of transcriptional and epigenetic programs in cancer cells using a broad unbiased cell-based screening strategy. Here, we report the identification of a chemical modulator, named JIB-04, which, using a novel mechanism, inhibits the demethylase activity of Jumonji enzymes in vitro and in cells, without affecting other α-ketoglutarate-dependent hydroxylases or histone-modifying enzymes. JIB-04 alters transcriptional growth programmes in cancer but not in normal cells, leading to cancer-specific cell death. Importantly, in vivo , JIB-04 lowers histone demethylase activity in tumours, reduces tumour burden and prolongs cancer survival in mice. Thus, we report the discovery and characterization of a novel, specific small-molecule inhibitor of the Jumonji enzymes, which is cell permeable, lowers histone demethylase activity in cultured cancer cells and in tumours, and exhibits selective anticancer properties in vitro and in vivo . Identification of a small molecule with epigenetic activity As tumours have an aberrant epigenetic landscape, the cancer epigenome must have unique susceptibilities that can be chemically targeted. We therefore developed a cell-based assay to identify small-molecule epigenetic modulators with potential anticancer properties. The system, named locus derepression (LDR), consists of mammary adenocarcinoma cells containing a stably integrated GFP–oestrogen receptor transgene driven by the CMV promoter, which is subject to epigenetic regulation. The GFP construct is repressed under standard growth conditions, but is induced by known epigenetic modulators, such as HDAC inhibitors ( Supplementary Fig. S1a ), but not by general activators of transcription, growth or stress [24] , [25] . Using automated fluorescence microscopy [26] , [27] , we first queried the NCI’s diversity set (a structurally diverse library of 2,080 compounds) to identify activators of the expression of the GFP fusion protein in our system. Among other hits [24] , NSC693627 (ref. 28 ), a pyridine hydrazone named JIB-04 shown in Fig. 1a , induced GFP dose-dependently ( Fig. 1b ). As JIB-04 has two forms, we synthesized and evaluated the activity of the pure E- versus Z-isomers. Only the E-isomer was active in the LDR assay ( Fig. 1a ). The active form of JIB-04 induced the transgene message and its action required de novo transcription, as actinomycin D abolished GFP production ( Fig. 1c ). Unlike the GFP inducer trichostatin A, however, JIB-04 did not inhibit HDACs ( Fig. 1e and Supplementary Fig. S1 ). We, therefore, identified JIB-04 E-isomer (hereafter, referred simply as JIB-04 or as E-isomer) as a transcriptional modulator that induced the expression of a silenced transgene without affecting HDACs. 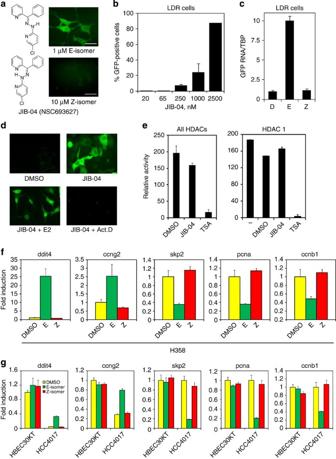Figure 1: Identification of a small molecule that modulates transcription in a cancer-selective manner. (a) The structure of JIB-04 E (top) and Z (bottom) isomers (NSC693627) and their activity on LDR cells as measured by fluorescence microscopy. Scale bars represent 50 μm. (b) Dose response of GFP induction by JIB-04 as measured by FACS analysis. (c) Only E-isomer JIB-04 increases GFP RNA levels in LDR cells. D, DMSO; E, 1 μM E-isomer; Z, 1 μM Z-isomer. (d) GFP induction in LDR cells by JIB-04 requires active transcription. LDR cells were treated with DMSO, 1 μM JIB-04±0.1 μM oestradiol (E2), or 0.5 μg ml−1Actinomycin D. Oestradiol induces nuclear translocation of the GFP-oestrogen receptor construct confirming fluorescent signal is not a false positive. (a–d) All cell treatments were overnight. (e) JIB-04 does not inhibit HDAC activity in cell lysates (left panel) nor in purified systems (right panel). 5 μM JIB-04 treatments are shown. (b,c,e) Mean+s.d. are shown from two independent experiments in (b) and from triplicates in (c) and (e). (f) Isomer-specific gene expression changes in growth control genes in H358 cells measured by qRT-PCR. (g) JIB-04 upregulates anti-growth genes and downregulates pro-growth genes in cancer, but not in normal matched cells. Expression is normalized to HBEC DMSO (up genes) or to DMSO for each cell line (down genes). (f,g) Mean across triplicates+s.d. of fold change are shown. 500 nM E or Z JIB-04 for 24 h was used. Figure 1: Identification of a small molecule that modulates transcription in a cancer-selective manner. ( a ) The structure of JIB-04 E (top) and Z (bottom) isomers (NSC693627) and their activity on LDR cells as measured by fluorescence microscopy. Scale bars represent 50 μm. ( b ) Dose response of GFP induction by JIB-04 as measured by FACS analysis. ( c ) Only E-isomer JIB-04 increases GFP RNA levels in LDR cells. D, DMSO; E, 1 μM E-isomer; Z, 1 μM Z-isomer. ( d ) GFP induction in LDR cells by JIB-04 requires active transcription. LDR cells were treated with DMSO, 1 μM JIB-04±0.1 μM oestradiol (E2), or 0.5 μg ml −1 Actinomycin D. Oestradiol induces nuclear translocation of the GFP-oestrogen receptor construct confirming fluorescent signal is not a false positive. ( a – d ) All cell treatments were overnight. ( e ) JIB-04 does not inhibit HDAC activity in cell lysates (left panel) nor in purified systems (right panel). 5 μM JIB-04 treatments are shown. ( b , c , e ) Mean+s.d. are shown from two independent experiments in ( b ) and from triplicates in ( c ) and ( e ). ( f ) Isomer-specific gene expression changes in growth control genes in H358 cells measured by qRT-PCR. ( g ) JIB-04 upregulates anti-growth genes and downregulates pro-growth genes in cancer, but not in normal matched cells. Expression is normalized to HBEC DMSO (up genes) or to DMSO for each cell line (down genes). ( f , g ) Mean across triplicates+s.d. of fold change are shown. 500 nM E or Z JIB-04 for 24 h was used. Full size image JIB-04 modulates transcription in a cancer-selective manner To define more generally the transcriptional pathways specifically altered by the active isomer of JIB-04 in human cancer cells, gene expression profiling was performed on Illumina microarrays. Within 4 h of drug treatment, >100 genes were upregulated greater than two-fold by the E-isomer, but not by the Z-isomer, in H358 non-small cell lung cancer cells (NSCLC), and ~20 genes were downregulated ( Supplementary Data 1 and Fig. 1f ). Pathway and gene ontology analysis pointed to the upregulation of genes involved in negative regulation of proliferation, in cell death, in energy-deprivation responses and in glycolytic metabolism. Gene expression profiles after 24-h treatment showed the isomer-specific downregulation of the major factors of mitotic cell division ( Supplementary Data 2 ). Thus, the E- but not the Z-isomer of JIB-04 modulated the transcriptional output of cancer cells, affecting growth pathways. Remarkably, we found that most of the genes that were up- or downregulated by E-isomer in cancer cells were unaltered by the drug in patient-matched normal cells, as shown by microarray gene expression profiles and qRT-PCR validation in the HCC4017 NSCLC versus the patient-matched human bronchial epithelial 30KT (HBEC30KT) line ( Supplementary Data 1 and 2 and Fig. 1g ). Of interest, very few expressed genes were modulated by JIB-04 in normal cells compared with that in cancer cells ( Supplementary Data 1 and 2 ). Taken together, we concluded that the active E-isomer induced cancer-specific transcriptional changes. Striking examples include the downregulation of proliferative genes such as CCNB1, PCNA and the oncogene SKP2, and the upregulation of the antiproliferative/pro-apoptotic genes DDIT4 and CCNG2 ( Fig. 1f ). JIB-04 inhibits Jumonji demethylase activity in vitro Bioinformatic analysis of JIB-04-induced gene expression changes performed using the Connectivity Map tool (which contains a collection of gene expression signatures in response to >1,000 different perturbagens at www.broadinstitute.org/cmap/ ), uncovered similarities between the signature obtained with active JIB-04 and those described for the HDAC inhibitors TSA and vorinostat, the iron chelator deferoxamine (DFO), and the prolyl hydroxylase inhibitor dimethyloxalylglycine (DMOG). As JIB-04 did not inhibit HDACs ( Fig. 1e and Supplementary Fig. S1 ), we tested if these two other activities could mimic JIB-04-induced phenotypes, but they did not. DFO and DMOG, however, are both inhibitors of iron-dependent, α-ketoglutarate-dependent enzymes, by general iron chelation and co-substrate competition, respectively. This suggested the Jumonji C family of histone demethylases as potential targets of JIB-04. These iron- and α-ketoglutarate-dependent enzymes use molecular oxygen to hydroxylate lysines on histone substrates, and are amenable to inhibition by small molecules. It has been demonstrated that their enzymatic activity is not curtailed in moderate hypoxia [29] , differentiating them from the oxygen-sensing HIF prolyl hydroxylases. We directly tested the possibility that JIB-04 may target Jumonji family members by measuring its effect on the demethylase activity of recombinant JMJD2E (also known as KDM4E) on a trimethylated H3K9 peptide [17] , [18] . We observed strong inhibition of enzymatic activity, in the presence of the E- but not the Z-isomer ( Fig. 2a ), with no effect on the coupled formaldehyde dehydrogenase reaction used for quantification of the formaldehyde by-product, which yields fluorescent NADH ( Fig. 2a , E(FDH) bar). Furthermore, the demethylase activity of another family member, JMJD2D (KDM4D), was also specifically inhibited by JIB-04 E-isomer as measured by direct western analysis of a full-length histone substrate ( Fig. 2b , left panel). NMR experiments also confirmed that JIB-04 strongly inhibited JMJD2A (KDM4A) demethylase activity ( Fig. 2b , right panel). Thus, three distinct methods indicated JIB-04 may be a pan inhibitor of Jumonji histone demethylases. 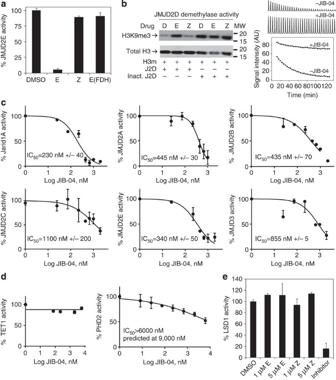Figure 2: JIB-04 specifically inhibits Jumonji histone demethylasesin vitroin a dose-dependent manner. (a) E-isomer-specific inhibition of JMJD2E enzymatic activity measured by formaldehyde release and downstream production of NADH, with no effect on the coupled formaldehyde dehydrogenase (FDH) reaction. Isomers were tested at 10 μM. (b) Direct measure of histone demethylation by western analysis (left panel, JMJD2D) and by NMR (right panel, JMJD2A) confirms inhibition of Jumonji enzyme activity by JIB-04. Left panel: J2D, JMJD2D; Inact J2D, heat-inactivated JMJD2D, E and Z at 2 μM. Right panel: expansions containing the trimethyl signal of the H3K9me3 peptide at 3.06 ppm in1H NMR spectra acquired as a function of time and plots of the time dependence of the intensity are shown. (c) Dose-response curves of JIB-04 inhibition across Jumonji demethylases measured by ELISA. Averages of 2–5 independent experiments are shown, with s.e.m. IC50values are given ±s.e.m. across separate experimental determinations;n=3 for JMJD2A,n=2 for JMJD2B,n=2 for JMJD2C,n=2 for JMJD2E,n=2 for Jarid1A,n=2 for JMJD3,n=5 for JMJD2DE. coli(Supplementary Fig. S2),n=2 for JMJD2D Sf9 (Supplementary Table S1). (d) JIB-04 selectively inhibits Jumonji enzymes over other cellular hydroxylasesin vitro. Mean of duplicates (TET1) or triplicates (PHD2) are shown, with s.e.m. (e) LSD1 enzymatic activity measured using purified recombinant protein in the presence or absence of JIB-04 isomers or positive control inhibitor. Error bars represent s.d. across duplicates from a representative experiment. Figure 2: JIB-04 specifically inhibits Jumonji histone demethylases in vitro in a dose-dependent manner. ( a ) E-isomer-specific inhibition of JMJD2E enzymatic activity measured by formaldehyde release and downstream production of NADH, with no effect on the coupled formaldehyde dehydrogenase (FDH) reaction. Isomers were tested at 10 μM. ( b ) Direct measure of histone demethylation by western analysis (left panel, JMJD2D) and by NMR (right panel, JMJD2A) confirms inhibition of Jumonji enzyme activity by JIB-04. Left panel: J2D, JMJD2D; Inact J2D, heat-inactivated JMJD2D, E and Z at 2 μM. Right panel: expansions containing the trimethyl signal of the H3K9me3 peptide at 3.06 ppm in 1 H NMR spectra acquired as a function of time and plots of the time dependence of the intensity are shown. ( c ) Dose-response curves of JIB-04 inhibition across Jumonji demethylases measured by ELISA. Averages of 2–5 independent experiments are shown, with s.e.m. IC 50 values are given ±s.e.m. across separate experimental determinations; n =3 for JMJD2A, n =2 for JMJD2B, n =2 for JMJD2C, n =2 for JMJD2E, n =2 for Jarid1A, n =2 for JMJD3, n =5 for JMJD2D E. coli ( Supplementary Fig. S2 ), n =2 for JMJD2D Sf9 ( Supplementary Table S1 ). ( d ) JIB-04 selectively inhibits Jumonji enzymes over other cellular hydroxylases in vitro . Mean of duplicates (TET1) or triplicates (PHD2) are shown, with s.e.m. ( e ) LSD1 enzymatic activity measured using purified recombinant protein in the presence or absence of JIB-04 isomers or positive control inhibitor. Error bars represent s.d. across duplicates from a representative experiment. Full size image To examine the potency and specificity of JIB-04 across Jumonji enzymes, we utilized a sensitive ELISA assay to directly quantify the demethylated histone substrate. Purified Jumonji demethylases representing several subfamilies were tested under equivalent conditions and exhibited distinct sensitivities to JIB-04 in vitro , with JARID1A (KDM5A) being the most sensitive (IC 50 =230 nM) and JMJD3 (KDM6B) and JMJD2C (KDM4C) more resistant (IC 50 ~1 μM) ( Fig. 2c ). The IC 50 ’s covered a <10-fold range ( Supplementary Table S1 ), establishing that JIB-04 is, in fact, a pan-selective inhibitor of Jumonji enzymes. Among the JMJD2 (KDM4) subfamily, JMJD2D had the highest sensitivity ( Supplementary Fig. S2g and Supplementary Table S1 ). No inhibition of the mechanistically related TET enzymes was observed and prolyl hydroxylases were only weakly affected (IC 50 >6 μM, predicted at 9 μM), demonstrating a window of specificity for histone lysine hydroxylases ( Fig. 2d ). The activity of the amine oxidase LSD1 (also known as KDM1A), which demethylates histone lysines using a distinct chemistry requiring FAD, was likewise uninhibited by JIB-04 ( Fig. 2e ). Similarly, other epigenetic enzymes including sirtuins, aurora kinases, protein arginine methyl transferases and histone methyl transferases were also unaffected (data not shown). Compared to JIB-04, the in vitro α-ketoglutarate competitive inhibitor 2,4-pyridinedicarboxylic acid was about five-fold less potent in blocking JMJD2D activity ( Supplementary Fig. S2f ) with an IC 50 =1.4 (±0.3) μM. To explore the mechanism by which JIB-04 inhibited Jumonji demethylases, we conducted competition assays. We found that while this small molecule, unlike known Jumonji inhibitors, was not a competitive inhibitor of α-ketoglutarate ( Supplementary Fig. S2a ), it clearly appeared competitive with respect to iron and potentially to the histone substrate and showed properties of mixed inhibition towards α-ketoglutarate in our biochemical assay ( Supplementary Fig. S2b and c ; note that K m is changed but V max is predicted to not change in Supplementary Fig. S2c , yet mixed inhibition towards the histone substrate remains a possibility as a plateau is not reached). JIB-04 interacted with iron likely in the catalytic site, as demonstrated by identical IC 50 values in the presence of 120 nM exogenous iron in solution or in the absence of exogenously added iron ( Supplementary Fig. S2d and e ) and by the lack of inhibition of other iron-dependent enzymes ( Fig. 2d ). The IC 50 of JIB-04 inhibition of JMJD2D was not dependent on the iron concentration in solution at doses <400 nM, but was affected at higher iron doses ( Supplementary Fig. S2d,e,g ), suggesting that iron chelation may contribute to inhibition when high doses of free iron are present in the solution. Taken together, these results define JIB-04 as a pan-selective inhibitor of Jumonji methyl-lysine hydroxylases affecting histone methylation levels in vitro in a unique manner that is not competitive with α-ketoglutarate. JIB-04 blocks growth and Jumonji demethylase activity in cells As Jumonji demethylases are deregulated in cancer, we evaluated JIB-04’s anticancer potential. To determine the specificity of JIB-04 for cancer, and to measure its potency, we performed cell viability assays in a large panel of human lung cancer (LCa) cell lines and in primary or immortalized non-tumorigenic HBECs, as well as in prostate cancer, primary prostate stromal and prostate epithelial cells. The range of IC 50 values after 4 days of drug exposure spanned nearly three orders of magnitude, demonstrating that the compound was not generally toxic ( Fig. 3a ). Importantly, JIB-04 was consistently selective for cancer versus normal cells, demonstrated by the higher sensitivity of LCa and prostate cancer lines (with IC 50 as low as 10 nM) compared with HBECs and primary prostate stromal/prostate epithelial cells ( Fig. 3a ). More strikingly, two pairs of patient-matched cell lines each derived from the cancerous and normal lung, respectively, of the same individual, confirmed JIB-04’s specificity for cancer ( Fig. 3b , compare HBEC30KT to HCC4017 and HBEC34KT to HCC4018), not seen with the HDAC inhibitor, depsipeptide ( Supplementary Fig. S3a ). JIB-04 was taken up similarly by both cell types, and cancer cells adapted to HBEC growth conditions remained sensitive to the drug (data not shown). Tested breast cancer cells were also more sensitive to JIB-04 than normal breast cells ( Supplementary Fig. S3b ). Soft-agar colony formation studies in multiple cell lines confirmed that JIB-04 potently inhibited tumorigenicity by interfering with anchorage-independent growth ( Supplementary Fig. S3c ). The ability of JIB-04 E-isomer to inhibit cancer cell viability was not simply the result of chelation of free iron, as excess iron did not rescue cells from JIB-04 death, while it did neutralize the effects of DFO ( Supplementary Fig. S3d , top panel), in agreement with earlier in vitro results ( Supplementary Fig. S2d and e ). In addition, a cell-permeable general inhibitor of α-ketoglutarate-dependent enzymes, dimethyloxalylglycine (D1070), also inhibited cell viability, although with a 1000-fold lower potency and only 5-fold selectivity for cancer compared with JIB-04 ( Fig. 3e ). 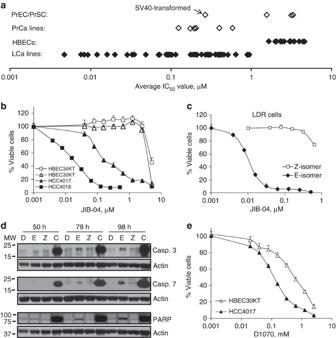Figure 3: JIB-04 E-isomer and its analogue have selective anticancer activity. (a) Log scale representation of cell viability IC50values comparing the sensitivities of unimmortalized and immortalized prostate (open symbol; PrEC/PrSC) or lung (closed symbol, HBEC) normal cells to prostate cancer (PrCa) or lung cancer (LCa) cells treated with JIB-04 over four days show JIB-04’s selective anticancer properties. (b) Cell viability dose response curves for patient-matched lines from normal and cancerous lungs treated with JIB-04 over four days confirm JIB-04’s cancer -specificity. Error bars represent s.d. across eight replicates. Compare HBEC30KT to HCC4017 and HBEC34KT to HCC4018. (c,d) The LDR active E-isomer but not the inactive Z-isomer potently inhibits LDR carcinoma cell viability (c) and induces apoptosis (d) as shown by the presence of cleaved caspase 3, 7 and PARP. (e) Cell viability dose response curves for one of the patient-matched pair of cell lines shown in (b) are given for dimethyloxalylglycine, D1070, a general inhibitor of α-ketoglutarate. Error bars represent s.d. across eight replicates. HCC4017 IC50=100 μM; HBEC30KT IC50=600 μM. Figure 3: JIB-04 E-isomer and its analogue have selective anticancer activity. ( a ) Log scale representation of cell viability IC 50 values comparing the sensitivities of unimmortalized and immortalized prostate (open symbol; PrEC/PrSC) or lung (closed symbol, HBEC) normal cells to prostate cancer (PrCa) or lung cancer (LCa) cells treated with JIB-04 over four days show JIB-04’s selective anticancer properties. ( b ) Cell viability dose response curves for patient-matched lines from normal and cancerous lungs treated with JIB-04 over four days confirm JIB-04’s cancer -specificity. Error bars represent s.d. across eight replicates. Compare HBEC30KT to HCC4017 and HBEC34KT to HCC4018. ( c , d ) The LDR active E-isomer but not the inactive Z-isomer potently inhibits LDR carcinoma cell viability ( c ) and induces apoptosis ( d ) as shown by the presence of cleaved caspase 3, 7 and PARP. ( e ) Cell viability dose response curves for one of the patient-matched pair of cell lines shown in ( b ) are given for dimethyloxalylglycine, D1070, a general inhibitor of α-ketoglutarate. Error bars represent s.d. across eight replicates. HCC4017 IC 50 =100 μM; HBEC30KT IC 50 =600 μM. Full size image In contrast to the E-isomer, the Z-isomer of JIB-04 was nearly 100-fold less potent in inhibiting cell viability ( Fig. 3c and Supplementary Fig. S3d , bottom panel). Cancer cells exposed to the E-isomer, but not the Z- isomer, underwent apoptotic cell death as evident at 48 h by Annexin V staining, caspases 3 and 7 activation and PARP cleavage ( Fig. 3d and Supplementary Fig. S3e ). The isomer-specific anti-growth activity, together with the isomer-specific activities observed earlier, indicated that the E-isomer acted through specific molecular interactions possibly blocked in the Z-isomer by the hydrogen bond formed by the pyridine nitrogen (compare the structures shown in Fig. 1a left panel), to inhibit Jumonji demethylases, alter transcription, and block cell growth. To explore this possibility, we synthesized a JIB-04 analog: an E-like symmetric molecule that leaves the nitrogen pyridine available for intermolecular interactions and a Z-like molecule that lacks the pyridine nitrogen ( Supplementary Fig. S3f ). The analog of E-isomer induced GFP in LDR cells, inhibited Jumonji activity in vitro and blocked cancer cell viability ( Supplementary Fig. S3f and g ). It also retained specificity for cancer versus normal cells, much like the parent compound ( Supplementary Fig. S3g , right most panel). In contrast, the analog of Z-isomer failed to induce GFP, to inhibit Jumonji activity in vitro and to block cell viability ( Supplementary Fig. S3f and g ). We thus concluded that JIB-04 targets cancer-specific susceptibilities in an isomer-selective manner that requires specific molecular interactions. To directly evaluate if JIB-04 affected histone demethylase activity in cells, we treated H358 NSCLC cells with DMSO, E- or Z-isomer and prepared soluble lysates, which we then tested for their ability to demethylate an H3K9me3 peptide substrate by detection of the H3K9me2 product. This assay allowed for the direct quantification of the demethylase activity of lysates on exogenous substrates, discounting indirect cellular drug effects that may lead to downstream changes in endogenous histone modifications. We observed a clear decrease in total H3K9me3 demethylase activity in lysates from cells treated with 0.1–2 μM E-isomer, but not with the inactive drug ( Fig. 4a ), establishing that JIB-04 inhibited H3K9me3 demethylases in cells at concentrations similar to the in vitro inhibition of individual purified enzymes ( Fig. 2c and Supplementary Table S1 ). No inhibition of HDAC activity was observed in these same cell lysates ( Supplementary Fig. S4a ), even at high JIB-04 doses. 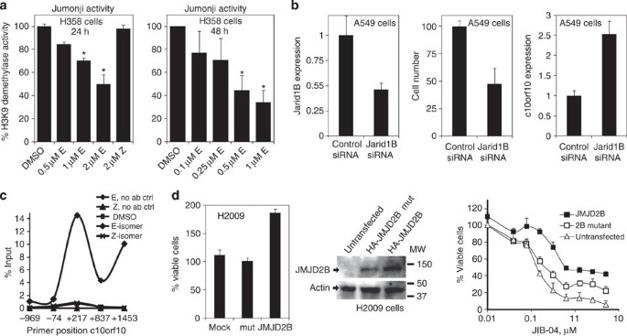Figure 4: JIB-04 inhibits cellular Jumonji demethylase activity, and Jumonji levels affect JIB-04 action in cells. (a) E-isomer lowers H3K9me3 demethylase activity in cancer cells dose-dependently. Activity is inhibited at lower doses of JIB-04 over prolonged exposure. Error bars represent s.e.m. across 2–3 independent assays. Asterisks denote statistically significant decreased activity of E-isomer versus DMSO-treated cells withP<0.05 for one-tailedt-tests. Cells were plated at five-times higher density than for standard viability assays to ensure sufficient surviving cells/enzymatic activity post drug treatment. (b) Knockdown of JARID1B (left panel) reduces cancer cell viability (middle panel) and increases c10orf10 expression (right panel), as does 4 h JIB-04 treatment (seeSupplementary Fig. S4). Error bars represent experimental error (left and right panels) or s.d. (middle panel) from the average of triplicates. (c) H3K4me3 levels are increased at the c10orf10 promoter in HCC4017 cells in response to treatment with 0.5 μM JIB-04 E-isomer for 24 h as measured by chromatin immunoprecipitation. (d) The increased basal viability of cells transiently overexpressing JMJD2B, but not the H189/E191Q JMJD2B mutant (mut), compared with mock-transfected cells (mock), is shown on the left panel. Overexpression of JMJD2B but not its mutant in H2009 lung cancer cells right shifts the response to JIB-04 (right panel). Averages across eight replicates are shown+s.d. The middle panel shows the expression levels of the HA-tagged wild type and mutant constructs for the cells in the right panel. Figure 4: JIB-04 inhibits cellular Jumonji demethylase activity, and Jumonji levels affect JIB-04 action in cells. ( a ) E-isomer lowers H3K9me3 demethylase activity in cancer cells dose-dependently. Activity is inhibited at lower doses of JIB-04 over prolonged exposure. Error bars represent s.e.m. across 2–3 independent assays. Asterisks denote statistically significant decreased activity of E-isomer versus DMSO-treated cells with P <0.05 for one-tailed t -tests. Cells were plated at five-times higher density than for standard viability assays to ensure sufficient surviving cells/enzymatic activity post drug treatment. ( b ) Knockdown of JARID1B (left panel) reduces cancer cell viability (middle panel) and increases c10orf10 expression (right panel), as does 4 h JIB-04 treatment (see Supplementary Fig. S4 ). Error bars represent experimental error (left and right panels) or s.d. (middle panel) from the average of triplicates. ( c ) H3K4me3 levels are increased at the c10orf10 promoter in HCC4017 cells in response to treatment with 0.5 μM JIB-04 E-isomer for 24 h as measured by chromatin immunoprecipitation. ( d ) The increased basal viability of cells transiently overexpressing JMJD2B, but not the H189/E191Q JMJD2B mutant (mut), compared with mock-transfected cells (mock), is shown on the left panel. Overexpression of JMJD2B but not its mutant in H2009 lung cancer cells right shifts the response to JIB-04 (right panel). Averages across eight replicates are shown+s.d. The middle panel shows the expression levels of the HA-tagged wild type and mutant constructs for the cells in the right panel. Full size image Jumonji enzyme levels modulate JIB-04 action in cells To evaluate whether the anti-proliferative action of JIB-04 could be the direct consequence of Jumonji enzyme inhibition, we knocked down a Jumonji H3K4me3 demethylase known to drive growth and measured LCa cell proliferation. Knockdown of JARID1B in LCa cells resulted in decreased viability and in higher expression of JARID1B target gene c10orf10 (refs 30 , 31 ), partly analogous to JIB-04 treatment ( Fig. 4b and Supplementary Fig. S4b and c ). Conversely, H3K4me3 levels were increased by JIB-04 on the promoter of this JARID1B target gene ( Fig. 4c ). On the other hand, overexpression of JMJD2B, but not an inactive H189G/E191Q demethylase mutant, resulted in higher basal viability compared with control cells ( Fig. 4d , left panel) and in decreased sensitivity to JIB-04 inhibition in LCa cells ( Fig. 4d , middle and right panels). This established that JIB-04’s transcriptional and anti-proliferative action is indeed, at least in part, directly the result of Jumonji inhibition. JIB-04 diminishes tumour growth in vivo To test if JIB-04 targeted cancer susceptibilities in vivo , we first generated and validated a large preparation of the E-isomer using a newly developed synthetic strategy ( Supplementary Fig. S5a ) and then evaluated its anticancer activity in two separate xenograft mouse models. H358 (whose viability in culture is inhibited by JIB-04 at 100 nM IC 50 ) or A549 (IC 50 =250 nM) LCa cells ( Supplementary Fig. S5b ), were injected subcutaneously into the flank of nude female mice and grown to 200 mm 3 . The drug was then administered 2–3 times weekly by IP injection at 110 mg kg −1 in sesame oil (H358 xenografts) or by gavage in Cremophor EL at 55 mg kg −1 to evaluate JIB-04’s oral efficacy (A549 xenografts). In all drug-treated animals, the rate of tumour growth was markedly diminished compared with that in the vehicle-treated cohorts ( Fig. 5a ). A significant decrease in final tumour weights was also observed in both models ( Fig. 5b ), with no effects on overall body weight or general health ( Fig. 5c ). Histological evaluation of major organs showed no abnormalities except for increased liver weights and liver vacuoles ( Supplementary Fig. S5c ). These results established that JIB-04 was effective in controlling LCa growth in animals whether given intraperitonealy or orally, and in two different formulations. 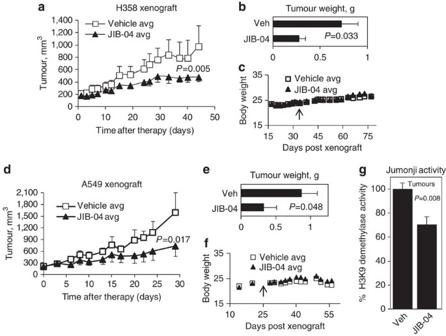Figure 5: JIB-04 diminishes tumour growth and inhibits tumour demethylasesin vivo. (a) H358 tumour growth is compromised in mice treated with E-isomer. Mean tumour volumes±s.e.m. (n=7 per group) are graphed across the 5-week treatment;P-value for the comparison of averages (one-tailedt-test) is shown. (b) Tumour burden is reduced in E-isomer-treated mice. Bars represent averages across groups+s.e.m. (n=7 per group);P-value across groups is given for a one-tailedt-test. (c) JIB-04 has no effect on body weight in H358 xenograft animals. (d–f) Tumour volumes, tumour weights and body weights are given for A549 tumour xenografts as above (n=7 per group). Arrows in (c) and (f) show start of treatment by IP injection or gavage, respectively. (g) JIB-04 E-isomer reduces H3K9me3 demethylase activity in tumoursin vivo. Error bars represent s.e.m. across three H358 and five A549 tumours per group;P-value across groups is given for a one-tailedt-test. Figure 5: JIB-04 diminishes tumour growth and inhibits tumour demethylases in vivo. ( a ) H358 tumour growth is compromised in mice treated with E-isomer. Mean tumour volumes±s.e.m. ( n =7 per group) are graphed across the 5-week treatment; P -value for the comparison of averages (one-tailed t -test) is shown. ( b ) Tumour burden is reduced in E-isomer-treated mice. Bars represent averages across groups+s.e.m. ( n =7 per group); P -value across groups is given for a one-tailed t -test. ( c ) JIB-04 has no effect on body weight in H358 xenograft animals. ( d – f ) Tumour volumes, tumour weights and body weights are given for A549 tumour xenografts as above ( n =7 per group). Arrows in ( c ) and ( f ) show start of treatment by IP injection or gavage, respectively. ( g ) JIB-04 E-isomer reduces H3K9me3 demethylase activity in tumours in vivo . Error bars represent s.e.m. across three H358 and five A549 tumours per group; P -value across groups is given for a one-tailed t -test. Full size image JIB-04 lowers Jumonji histone demethylase activity in tumours Having seen that the active E-isomer of JIB-04 inhibited H3K9me3 demethylases in vitro and in cells, and having established that this active isomer effectively reduced cancer growth in culture and in vivo , we next asked whether tumours from mice treated with JIB-04 had altered histone demethylase activity compared with tumours from vehicle-treated mice. Tumour lysates were therefore assayed for their ability to demethylate an exogenous H3K9me3 substrate to produce the H3K9me2 product. Remarkably, lysates of H358 and of A549 tumours from mice treated in vivo with JIB-04, showed reduced total H3K9me3 demethylase activity compared with tumours from vehicle-treated mice ( Fig. 5g ), while the HDAC activity in the same tumour lysates was unaffected ( Supplementary Fig. S5d ). Thus, the very same JIB-04-treated tumours that were significantly blunted in their growth in vivo (described in Fig. 5a–f ) also had significantly diminished Jumonji histone demethylase activity. JIB-04 prolongs cancer survival To further assess the in vivo efficacy of JIB-04, we evaluated the effect of JIB-04 on the survival of immune-competent BALB/c mice bearing orthotopic 4T1 mammary tumours. 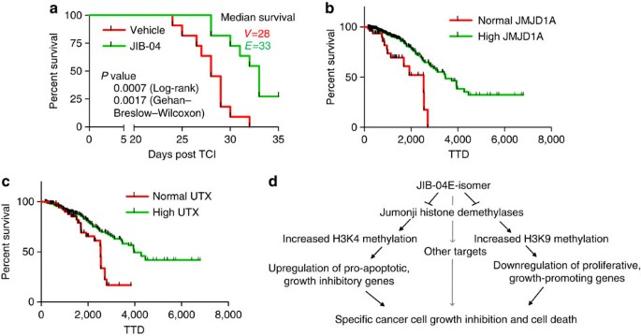Figure 6: JIB-04 prolongs cancer survival. (a) JIB-04 increases cancer median survival from 28 to 33 days in an aggressive 4T1 breast cancer model. Note that three animals in the drug-treated cohort were still alive at the end of the study;n=11 per group. (b,c) Human breast cancer patients with high levels of the indicated Jumonji enzymes have significantly worse prognosis. Hazard ratios are 3.1 for JMJD1A (95% CI: 1.7–5.6) and 2 for UTX (95% CI: 1.2–3.4). (d) Working model of the cancer-selective mode of action of JIB-04 E-isomer. Therapy with JIB-04, initiated in animals with established tumour burden, significantly extended survival compared with the matched vehicle-treated mice (median survival of 33 days versus 28 days, which is an 18% increase in lifespan post cancer onset), as shown in Figure 6a . Vehicle-treated mice had a hazard ratio of 7.3 over JIB-04-treated mice. This demonstrates that the anti-proliferative effects of JIB-04 in vivo result in a significant reduction in cancer-induced death rates in mice, prolonging survival. Of clinical importance, our analysis of The Cancer Genome Atlas (TCGA) human breast cancer data ( n =729) showed a significantly poorer survival and 2–3 times higher risk of death for patients bearing tumours that expressed high levels of the specified Jumonji enzymes compared with those expressing normal or low levels ( Fig. 6b ), defining a human subpopulation that may indeed benefit from an JIB-04-like intervention in the future. Figure 6: JIB-04 prolongs cancer survival. ( a ) JIB-04 increases cancer median survival from 28 to 33 days in an aggressive 4T1 breast cancer model. Note that three animals in the drug-treated cohort were still alive at the end of the study; n =11 per group. ( b , c ) Human breast cancer patients with high levels of the indicated Jumonji enzymes have significantly worse prognosis. Hazard ratios are 3.1 for JMJD1A (95% CI: 1.7–5.6) and 2 for UTX (95% CI: 1.2–3.4). ( d ) Working model of the cancer-selective mode of action of JIB-04 E-isomer. Full size image Here, we report the discovery of a novel pan-selective inhibitor of Jumonji demethylases that exhibits some selectivity in vitro for the H3K4me3 demethylases and the pure H3K9me3 demethylases over the H3K27 demethylases or mixed H3K9/H3K36 demethylases, but does not affect the activity of other histone-modifying enzymes. JIB-04 shows selective anticancer activity in cell culture across several tumour types and in vivo in mouse tumour xenografts, without general toxicity. Importantly, this small molecule increases cancer survival in an aggressive breast cancer model. JIB-04’s anti-proliferative effects are isomer-specific and are at least partly mediated through direct cancer-specific transcriptional changes in genes that control cell growth, resulting in tumour cell death. The compound lowers histone demethylase activity in vitro , in cultured cells and in tumours in vivo and can modulate histone methylation levels on target genes. To our knowledge, this is the first inhibitor of Jumonji enzymes with selective anticancer properties in vitro , in cells and in vivo . JIB-04 expands the chemical space where Jumonji inhibitors may be found, as it is structurally novel and not an analog of hydroxylase co-factors. The isomer chemistry and the overall structure of JIB-04 make it attractive for further structure–activity relationship studies of related molecules, which could be characterized for their ability to modulate particular Jumonji demethylase-dependent functions such as JMJD2A’s involvement in DNA replication [32] or the recently described role of JARID1A in the development of drug resistance [33] . As a whole, this study demonstrates how a broad, functionally meaningful screening system can lead to the identification of novel chemical activities and open up aspects of disease biology and cellular regulatory pathways that are therapeutically relevant, as demonstrated here by the population of human breast cancer patients we identified who have a 2–3 fold higher risk of death due to increased levels of Jumonji demethylase expression. The Jumonji family of histone demethylases has been the focus of much study over the last few years. Numerous reports have demonstrated the relevance of these enzymes in a variety of physiological and pathological conditions beyond cancer, including early development, reproduction, metabolism and cardiac hypertrophy [6] , [34] , [35] , [36] , [37] , [38] , [39] , [40] . The structure of Jumonji catalytic domains shows they are drugable [41] , [42] , [43] , able to accommodate small molecule disruptors, making them ideal molecular targets for intervention. Modulation of aberrant Jumonji demethylase activity in disease should lead to the normalization of transcriptional patterns, such as we see with JIB-04 in cancer cells. JIB-04’s ability to block tumour growth and prolong cancer survival may involve both direct and indirect aggregate effects of Jumonji enzyme pan-inhibition in cells and in vivo ( Fig. 6d ), and it is possible that the drug accumulates in cancer cells over time, increasing its effective concentration/apparent potency. Mechanistically, JIB-04 appears to chelate iron in the catalytic site of Jumonji enzymes and to disrupt histone substrate binding, while not being a competitive inhibitor for α-ketoglutarate, a mechanism not yet described for Jumonji inhibitors. Future structural information will be necessary to establish the exact molecular interactions between Jumonji enzymes and their co-factors/substrates that are disrupted by JIB-04. One possibility is that the inhibitor may occupy the outer portion of the active site where the iron and the histone substrate bind, or bind to iron in the active site in a manner that alters subsequent substrate binding [43] , [44] , [45] . Chelation in solution may also contribute to inhibition under conditions of high free iron. In vitro inhibitors of Jumonji demethylases have been described recently (refer to the study by Rose et al. [45] for an excellent review) and include analogs of α-ketoglutarate and structurally related series [16] , [17] , [18] , [19] , [20] , [21] , [22] with varying potencies in vitro and in some cases, cellular activity at high doses. Although these compounds are useful probes for further inhibitor development, none have been shown to have activity in vivo . Our small molecule is structurally distinct, combining pyridine moieties—which are known to contribute to the inhibition of related hydroxylases in the context of α-ketoglutarate mimics—and a hydrazone group that together give the compound nanomolar potency and cancer-specificity in cells. JIB-04 shows anticancer activity in two relevant preclinical animal cancer models by two routes of administration and increases cancer survival. The broad, unbiased screen for biological activity used here to identify JIB-04—in contrast to in vitro biochemical methods, for example—may indeed prove to be most effective in identifying pan-selective or specific inhibitors of disease pathways with activity in cells and in vivo . Thus, we propose that a biologically relevant strategy at the screening step, such as the one followed recently by GlaxoSmithKline [46] , [47] , may result in more effective drugs for any therapeutic application down the pipeline. A feature of cancer cells is their ability to sustain proliferation, trigger a pro-inflammatory and pro-invasive environment, deregulate energy pathways, and avoid growth inhibition, immune destruction and death signals [48] . In ways that are not yet fully understood, JIB-04 seems to curtail cancer survival by off-setting most of these tumour-promoting advantages. The compound downregulates growth-promoting genes, modulates genes involved in energy metabolism and makes cancer cells susceptible to death signals that it induces. Whether all or only a subset of these actions is mediated by Jumonji enzymes and their downstream targets is not yet fully clear. Precedent exists, however, for the involvement of Jumonji enzyme in all these processes, opening the way for therapeutic intervention in inflammatory, growth and metabolic disorders, also through the modulation of demethylase activity. Cell culture and viability assays Cancer cell lines (gifts from Drs John Minna, Cheryl Lewis and J.T. Hsieh, or purchased from ATCC) were maintained in RPMI media with 5% fetal bovine serum, unless otherwise specified. Human bronchial epithelial cells, unimmortalized or immortalized with cdk4 and telomerase, were cultured in KSFM media with EGF and pituitary extract (KSFM supplements from Gibco) [49] . Human mammary epithelial cells immortalized with telomerase were maintained in complete MEGM media from Cambrex. All cell lines were routinely tested for mycoplasma and fingerprinted. Cells were transfected with Lipofectamine 2000, following the manufacturer’s protocol. Expression vectors pCMV-HA-JMJD2B and pCMV-HA-JMJD2B-H189G/E191Q were kindly provided by Dr Jesper Christensen [50] . Cell viability was assessed by standard MTS assays using Promega’s Cell Titer or Cell Titer-Glo reagents. The average IC 50 derived from 2–5 independent assays, each containing 4–8 replicates, is reported. Further details about cell culture, transfections and viability assays are given in Supplementary Methods . Connectivity map queries Tags of genes up- or downregulated more than two-fold by compound treatment in the microarray gene expression data were converted to Affymetrix IDs and used to build signatures to query the Connectivity map database [51] at www.broadinstitute.org/cmap/ . This analysis scores the similarity between the query gene signature and catalogued signatures of up- and downregulated genes in response to known perturbations. Soft-agar colony formation 0.5% agar in RPMI supplemented with 20% FCS and antibiotics and containing increasing amounts of drug were poured and allowed to settle before adding a top 0.33% agar layer containing cells. Agar was kept moist with 0.5 ml of growth media containing drug or vehicle, changed 2–3 times per week. After 2–3 weeks, colonies (clusters greater than ~50 cells) were counted manually by two observers. The number of colonies in duplicate or triplicate wells per condition was averaged. Fluorescence microscopy GFP expression in LDR cells in response to drug treatments was monitored by fluorescence microscopy. Cells were plated on coverslip glass chambers (Labtek II, Nunc) and after 24 h were drug-treated overnight. Cells were washed, fixed with 4% paraformaldehyde and visualized under a Nikon Eclipse TE2000-U fluorescence microscope equipped with a CCD Roper camera. Images were processed under identical conditions with Metamorph software. FACS To quantify GFP expression, LDR cells were collected and resuspended in PBS at 100,000 cells per ml and subjected to FACs. Data were analyzed using FlowJo software. Uninduced and vehicle-treated cells were used as a negative control for gating. The Annexin V-FITC apoptosis detection kit I from BD Pharmingen was used for measurements of phosphatidylserine membrane flipping, per the manufacturer’s protocol. Unstained cells were used for gating. All samples were analysed in a BD FACSCalibur sorter. HDAC activity assays Cell extracts or purified recombinant HDAC enzymes were used in standard HDAC activity assays using Millipore’s HDAC Fluorometric Assay Kit, according to the manufacturer’s protocol, with vehicle or drugs. A FluoroStar Omega plate reader (BMG Biosciences) was used for fluorescent detection. Purified recombinant active HDACs were purchased from Millipore/Upstate. Synthetic chemistry Large-scale synthesis of total JIB-04, NSC693627, was carried out in our Synthetic Chemistry core at UTSW, following established procedures [28] . For the production of E-isomer (shown in Supplementary Fig. S5a ), please see Supplementary Methods . Mouse studies and in vivo drug administration For xenografts, 4–6-weeks-old female nude mice were used. For the survival study [52] , Balb/c 6–8-weeks-old female mice were utilized. Animals were housed under standard conditions in a clean facility at UTSW. All animal experiments were carried out under approved IACUC protocols and followed UTSW animal care procedures. Detailed in vivo protocols are given in Supplementary Methods . TCGA expression and survival data analysis Public clinical and RNA-Seq data of 729 patients of breast invasive carcinoma were obtained from TCGA portal ( https://tcga-data.nci.nih.gov/tcga ). The longest time the patients were followed up or known to be alive was considered for the survival analysis. Gene expression that was normalized with the reads per kilobase of exon model per million mapped reads method was obtained from the RNA-Seq data. A gene was considered to be upregulated in patients whose expression levels were one s.d. higher than the average of all patients. Gene upregulation was correlated with the overall survival using Kaplan–Meier tables and compared with the Log-rank test under SPSS Statistics 17.0. Hazard ratios were calculated using Cox regression. GraphPad Prism was used to represent data graphically. Histology Tissues were preserved in formalin at the time of harvest and submitted to the Pathology core at UTSW for histological sectioning and staining with H&E. Animals not bearing tumours, but subjected to 2 weeks of drug or vehicle treatment in parallel with xenografted animals under identical conditions, were used to monitor organ health and drug toxicity. Western blots Cancer cells treated as indicated were lysed in RIPA buffer, protein was quantified and equal amounts of protein run on 4–12% SDS acrylamide gels. Protein was transferred to nitrocellulose membranes and blotted for cleaved (activated) caspases 3 (Cell Signaling #9661 at 1:1,000 dilution), 7 (Cell Signaling #9491 at 1:1,000), 8 (Santa Cruz 5263 at 1:200), 9 (Cell Signaling #9501 at 1:800), 10 (Calbiochem PC332 at 1:1,000), cleaved PARP (#9541 at 1:1,000), or HA-tag (clone 3F10, Roch #11867423001 at 1:3,000). Bands were imaged using enhanced chemiluminescence reagents from Thermo Scientific. Microarray gene expression profiles and pathway analysis RNA was extracted using the RNeasy kit (Qiagen) and quality was evaluated with the Experion gel system (BioRad), prior to labeling at UTSW’s microarray core. Labelled RNA was hybridized to Illumina human WG6 version 2 (H358) or version 3 (matched pair) microarray chips according to the manufactor’s protocol. All genes on the arrays were verified by BLAST and annotated using recent versions of public NCBI databases. Microarray analysis was done with BeadStudio 3 and in-house Visual Basic software MATRIX 1.33. Array data were quantile-normalized and samples were compared by calculating log 2 ratios for each gene along with a t -test P -value. Functional relationships were analysed with the Ingenuity Pathway gene annotation software. The microarray gene expression data and gene annotations can be retrieved from the Supplementary Information , Supplementary Data 1 and 2 . Quantitative RT-PCR reactions and data analysis RNA was extracted with RNeasy technology (Qiagen), quantified, DNAse-treated and reverse-transcribed. The cDNA was then amplified with Sybr green chemistry in real-time quantitative PCR assays (Applied Biosystems) using validated primers. Reactions were performed on an ABI Prism 7900HT. The data were analysed with the ddCt method as previously described [53] . Primer sequences and further details are given in Supplementary Methods . Jumonji demethylase/prolyl hydroxylase/TET/LSD1 activity assays Active JMJD2E aa 1-350 was purified from Escherichia coli and used in vitro in a coupled reaction as previously described [18] or using Epigentek kit P-3081. For histone demethylation reactions quantified by western analysis, a His-tagged hJMJ2D aa 1-350 expression construct, the kind gift of Drs Y. Shi and J. Whetstine, was expressed and purified from E. coli following the Qiagen Ni-NTA agarose manual instructions and the protocol of Whestine et al. [54] For in vitro IC 50 determination and competition studies, typically 100–200 ng of purified protein (as above, or purchased from BPS Bioscience catalog# 50110, 50111, 50105, 50117, 50118, 50115) was incubated with vehicle, JIB-04 or analogs, as indicated in the figure legends, and activity measured by ELISA (Epigentek kit P-3081). hJMJD2A (aa1-350) purified in E. coli [43] was the kind gift of Dr Jose Rizo-Rey and was assayed at 400 ng per reaction due to its intrinsic low activity. GraphPad Prism software was used for IC 50 calculations and curve fitting. Full details of all demethylase activity assays and of the prolyl hydroxylase reactions are given in Supplementary Methods . The activity of LSD1 recombinant protein (a gift of Dr Chen-Ming Chiang) was measured using Epigentek kit P-3075 according to the manufacturer’s protocol. TET1 activity (Active Motif #31363) was measured using Epigentek P-3087. NMR 1 H NMR experiments were performed at 25 °C and 600 MHz on an Agilent INOVA spectrometer equipped with a cold probe. Samples contained 35 μM JMJD2A and 160 μM 2-OG, dissolved in 25 mM Tris, pH 7.4, 125 mM NaCl, 5% D8-Glycerol and 1 mM TCEP buffer (8% D 2 O). For experiments performed in the presence of JIB-04, the compound was dissolved in DMSO-d 6 and added to the NMR sample to a nominal final concentration of 160 μM. The spectra were acquired with a Carr–Purcell–Meiboom–Gill sequence applied for 0.1 ms before the acquisition time to relax the protein signals and allow better observation of the peptide signals. Please see Supplementary Methods for full details. Chromatin immunoprecipitations Chromatin immunoprecipitation experiments were carried out following the Millipore ChIP Assay Kit protocol (Millipore, #17-295). Briefly, exponentially growing matched pair cells were crosslinked after drug treatment in 1% formaldehyde for 10 min at 37 °C. Chromatin was isolated and sheared, and immunoprecipitated using 2 μg of α-H3K4me3 antibody (Millipore, #07-473) or no antibody control. Crosslinking was reversed at 65 °C for 4 h with 200 mM NaCl. DNA was isolated and purified using the QIAquick PCR Purification Kit (Qiagen, #28106). The presence of DNA associated with the pulled down H3K4me3 was quantified through qPCR as described above and expressed as percent input. Primers used to scan the promoter and into the coding region are listed in Supplementary Methods . Statistical analysis Statistical analysis was carried out as stated in each figure/legend and further detailed in the corresponding methods sections. Briefly, P -values were calculated using Student t -tests (Excel), log-rank, or Gehan–Breslow–Wilcoxon (GraphPad Prism), as indicated, and hazard ratios were calculated using Cox regression (SPSS Statistics 17.0). Error bars are defined in each figure legend. Accession codes: Microarray data have been deposited in the National Center for Biotechnology Information Gene Expression Omnibus database under accession code GEO46632 . How to cite this article: Wang, L. et al. A small molecule modulates Jumonji histone demethylase activity and selectively inhibits cancer growth. Nat. Commun. 4:2035 doi: 10.1038/ncomms3035 (2013).